Representational format determines numerical competence in monkeys A range of animal species possess an evolutionarily ancient system for representing number, which provides the foundation for simple arithmetical operations such as addition and numerical comparisons. Surprisingly, non-human primates tested in ecologically, highly valid quantity discrimination tasks using edible items often show a relatively low performance, suggesting that stimulus salience interferes with rational decision making. Here we show that quantity discrimination was indeed significantly enhanced when monkeys were tested with inedible items compared with food items (84 versus 69% correct). More importantly, when monkeys were tested with food, but rewarded with other food items, the accuracy was equally high (86%). The results indicate that the internal representation of the stimuli, not their physical quality, determined performance. Reward replacement apparently facilitated representation of the food items as signifiers for other foods, which in turn supported a higher acuity in decision making. The ability to judge quantities is of great relevance in a variety of ecological contexts, such as predation, foraging and breeding [1] . Previous research conducted in the laboratory and in the field has provided compelling evidence that numerical abilities are not exclusively human (for reviews see refs [2] , [3] ). Some basic arithmetical skills have been shown in dogs [4] , cats [5] , chicks [6] and even mosquitofish ( Gambusia holbrooki ) [7] , suggesting that a broad array of species possesses an evolutionarily ancient system for representing numbers. On the assumption that food quantity discrimination is ecologically highly valid, numerical skills of animals have frequently been examined through testing whether they are able to select the larger of two food quantities (relative numerousness judgment) [8] , [9] , [10] , [11] . A further advantage of using food quantity discrimination is that it avoids complicated or time-consuming training procedures, which must be employed when symbols are used [12] , [13] . Somewhat counter-intuitively, however, studies using simple food quantity discrimination paradigms often report performance at relatively low levels. Western lowland gorillas ( Gorilla gorilla gorilla) , for instance, performed at chance level in a food quantity discrimination task and only learned to select the larger of two food quantities after additional training [14] . Similarly, chimpanzees and orang-utans performed only at ∼ 65% correct in a relatively simple food quantity discrimination task [15] . But why is this the case? From reversed reward paradigms it is known that the salience of the choice stimulus is a crucial factor in experiments. In this paradigm, animals have to point to the smaller quantity to obtain the larger one. Chimpanzees fail at this task, as they appear to be unable to inhibit reaching towards the larger food amount. In contrast, when symbols (Arabic numerals) were used, they did significantly better [16] . To gain a better understanding of the factors that support accurate decision making, we tested Old World monkeys in a series of quantity discrimination tasks. We conducted two-choice experiments with olive baboons ( Papio anubis ) and long-tailed macaques ( Macaca fascicularis ), in which they had to discriminate between arrays of edible and inedible items (pebbles). We predicted that the monkeys would perform better when tested with inedible, that is, less salient items. There are two possible explanations. For one, the highly salient food items might impair impulse inhibition. Alternatively, the monkeys might have difficulties to simultaneously maintain two mental representations of the food items, first as choice stimulus and second as food reward [17] . To distinguish between these two possible explanations, we introduced a third condition in which the monkeys were required to discriminate between food items, but under a different reward contingency scheme: in this experiment, the monkeys were not rewarded with the food items they had pointed at, but with other food items of the same kind as the choice stimuli hidden underneath the plates presenting the food. Our results revealed that the reward contingency is more important than stimulus salience, as subjects performed equally well when tested with inedible items and when food items were replaced. These findings suggest that the mental representation of what choice stimuli stand for is more important for controlling choice behaviour than physical appearance of the stimuli. Procedure We tested 16 Old world monkeys (olive baboons and long-tailed macaques) housed at the German Primate Center in a two-choice paradigm. Animals were presented simultaneously with two different amounts (1–8 items) of edible (raisins or peanuts) or inedible items (pebbles). 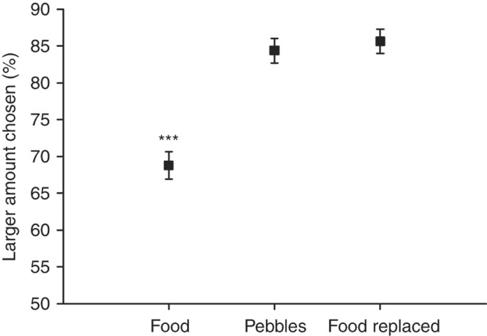Figure 1: Percent of trials in which the larger quantity was chosen in the different test conditions (means and standard error of means). Performance in the 'Food' condition was significantly worse than in the other two conditions (GLMM,N=16 subjects;P<0.001). Quantities differed in magnitude from 1 to 4 ( Table 1 ). After the subjects made their choice by pointing at the desired quantity, they were rewarded either with the food items they had pointed at or with an amount of food equivalent to the amount chosen. To accustom the monkeys to the respective choice paradigm, they passed a short familiarization phase before the actual test phase of each condition began. 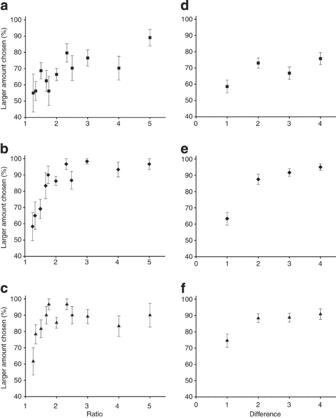Figure 2: Effects of relative and absolute difference between choice stimuli on performance. Percent of trials in which the larger amount was chosen (means and standard error of means) in relation to the ratio between the quantities presented for the three different conditions (a) Food, (b) Pebbles, (c) Food replaced; and in relation to the absolute difference between quantities (d) Food, (e) Pebbles, (f) Food replaced. There was a combined effect of relative and absolute difference on performance (GLMM,N=16 subjects, Effect of absolute differenceP=0.0001, Effect of ratioP=0.0024). There was no significant difference in performance between the two species across conditions (generalized linear mixed model (GLMM) analysis with Monte-Carlo-Markov chain (MCMC) procedure: N =16, P =0.25, Table 2 ); therefore, results are presented for the pooled data set. Table 1 Absolute difference and ratios of the quantities used in the experiments. Full size table Table 2 Effects of the different predictor variables on performance. Full size table Test conditions In the ecologically most valid 'Food' condition, food items were used as choice stimuli and as rewards; that is, the food items selected by the monkey were fed to her ( Supplementary Movie 1 ). In this condition, the monkeys chose the larger amount above chance but at relatively low levels (68.8% of the choices; Fig. 1 ). When small black pebbles served as choice stimuli, and the animals were rewarded with the equivalent amount of food items (Pebble condition), subjects chose the larger amount of items significantly more frequently (84.4%; Fig. 1 , Table 2 ; N =16; post hoc test between these two conditions: P <0.001). Figure 1: Percent of trials in which the larger quantity was chosen in the different test conditions (means and standard error of means). Performance in the 'Food' condition was significantly worse than in the other two conditions (GLMM, N =16 subjects; P <0.001). Full size image In the 'Food replaced' condition, the subjects were rewarded with other food items hidden underneath the plates presenting the food. In this condition, the choice stimulus was highly salient, while choice stimulus and reward were separate entities, that is, the reward contingency was the same as in the non-food condition. If the performance of the monkeys is determined by the quality of the stimulus (being edible or not), they should obtain similar poor results in the Food and 'Food replaced' conditions. In contrast, if the reward contingency is decisive, they should do well both when tested with inedible items and when rewarded with other food items. In this condition, the subjects performed at a similar level as in the 'Pebbles' condition (see Fig. 1 , post hoc test: P =0.59) and significantly better than in the initial 'Food' condition ( Supplementary Movie 2 ). They chose the larger amount in 85.6% of all trials ( post hoc test: P <0.001). The performance of the animals in all three conditions was influenced by the absolute magnitude of the difference between the two quantities as well as the ratio between the two quantities (GLMM analysis with MCMC procedure, Fig. 2 and Table 2 ). Figure 2: Effects of relative and absolute difference between choice stimuli on performance. Percent of trials in which the larger amount was chosen (means and standard error of means) in relation to the ratio between the quantities presented for the three different conditions ( a ) Food, ( b ) Pebbles, ( c ) Food replaced; and in relation to the absolute difference between quantities ( d ) Food, ( e ) Pebbles, ( f ) Food replaced. There was a combined effect of relative and absolute difference on performance (GLMM, N =16 subjects, Effect of absolute difference P =0.0001, Effect of ratio P =0.0024). Full size image Control conditions To test the hypothesis that the poor performance in the Food condition was due to the changing appearance of the choice stimuli while the food items were given to the monkeys, leading to a decrease in associative strength of these stimuli, we added two types of control conditions. Varying the appearance of the stimuli by either removing all food stuffs before giving them to the monkeys, or by removing a pebble each time one food item was given to the subject did not change the pattern: monkeys were still significantly better when discriminating between different amounts of pebbles (86% correct) compared with food items (75% correct; P <0.001). To test whether unintentional cueing by the experimenter might have affected the monkeys' performance ('Clever Hans effect'), we ran an additional control. In these experiments, we used boxes with a lid that opened to one side and small drawers to deposit the corresponding amount of food pieces. The boxes were baited by a second experimenter so that the first experimenter did not know how many pebbles were in each box. She then presented the boxes to the subjects and opened the lids so that the monkeys could see the content of the boxes while the experimenter could not. After choosing, the monkeys were rewarded with the food items in the corresponding box. There were no significant differences in performance in relation to whether the monkeys were tested in the regular 'Pebbles' condition or in the 'Experimenter blind' condition (mean±s.e.m. performance in the regular condition 0.81±0.03 and 0.81±0.02 in the Experimenter blind condition; T =10.5, N =8, P =1; exact Wilcoxon signed-ranks test). In the ecologically most valid 'Food' condition, the monkeys chose the larger amount above chance but at relatively low levels. In contrast, subjects chose the larger amount of items significantly more frequently in the 'Pebbles' condition. Thus, the monkeys' poor performance in the 'Food' condition was not due to an inability to discriminate between the different quantities. These results are compatible with the notion that highly salient stimuli impair impulse inhibition. Likewise, human children performed significantly better when symbolic representations substituted for real candies in the reversed-reward paradigm [18] , similar to the results obtained with chimpanzees [16] . Strikingly, in the critical 'Food replaced' condition, the subjects performed at a similar level as in the 'Pebbles' condition and significantly better than in the initial 'Food' condition. This finding refutes the assumption that a lack of impulse inhibition is the sole explanation for the poor performance in the 'Food' condition (see also ref. 19 for alternative explanations of the reversed-reward paradigm). Instead, the internal representation of the choice stimuli, not their physical quality, seems to be crucial for the improved performance. In particular, it appears that the monkeys fail to master the dual representation of the stimuli as choice stimulus and as food reward. 'Dual representation', that is, the mental representation of an object as well as the representation of the relation between an object and what it stands for, is seen as a foundation of abstract reasoning and symbolic understanding [17] . Research on children has shown that increasing the salience, that is, attractiveness of an object, impairs dual representation [17] . Our results suggest that in the 'Food' condition, our subjects failed at this dual representation, in the sense that they were unable to simultaneously maintain both representations of the items as food and as choice stimuli. In the 'Food replaced' condition, in contrast, the representation as food was diminished and that as signifiers for different quantities enhanced. This in turn supported the increase in accuracy. Representing food items as choice stimuli can be seen as a form of representational redescription (RR). RR is posited as a process by which implicit information in the mind becomes explicit knowledge to the mind by recoding information from one representational format to another [20] . Thus, the stimuli become available to explicit reasoning and decision making. Clearly though, this elementary form of RR needs to be distinguished from relational RR as described by Penn and colleagues [21] . Relational RR involves structurally systematic, rule-governed relational redescriptions, and, has been suggested to be a distinguishing feature of humans. Overall, the performance of our subjects was comparable with those of other monkey species [22] , [23] and great apes [15] . Their accuracy was influenced by the absolute magnitude of the difference as well as the ratio between the two quantities. Two different mechanisms have been invoked to account for numerousness judgments, the analogue magnitude and the object-file model (for a review, see for example, ref. 24 ). The analogue magnitude model estimates large numerical magnitudes and is characterized through (1) less accurate discrimination as the size of quantities increases and (2) as the ratio between the larger divided by the smaller magnitude decreases (Weber's law) [25] . The object-file model predicts a decline in discrimination ability when more than four items are to be judged. It operates by keeping track of individual objects and therefore serves for the representation of small exact numerosities. A range of studies found support for the analogue magnitude model [26] , [27] , whereas others favoured the object-file model [28] . Our results are in line with the assumptions of the analogue magnitude model, because performance was poor when the ratio approached 1. In contrast, the results are not compatible with the object-file model because subjects were still very good at discriminating between large quantities, for example, 7 and 3 items, and showed poor performance when the difference was small. Our results have two main implications. First, we demonstrate that quantity discrimination paradigms using food may underestimate the true competence of a species [29] . Second, we provide further insight into the conditions that favour rational decision making, specifically the effects of reducing the appetitive value of the choice stimulus. Taken together, our findings mirror those made with children [17] and suggest that the basic cognitive operations that facilitate abstract reasoning have deep evolutionary roots (see also refs [30] , [31] ). Subjects Six olive baboons ( Papio anubis )—four males and two females aged 3–9 years—living in a group of 11 animals and 10 long-tailed macaques ( Macaca fascicularis )—five males and five females aged 1–7 years—living in a group of 32 animals were tested. The animals were housed at the German Primate Center in Göttingen and had access to indoor (baboons: 17 sqm, macaques: 40 sqm) and outdoor areas (baboons: 81sqm, macaques: 141 sqm). They were individually tested in their familiar indoor cages. Water was always available ad libitum and subjects were not food deprived for testing. Materials Two round white plastic plates (height 0.01 m, diameter 0.08 m) were baited with different amounts of food items, that is, raisins or pieces of peanuts (one piece corresponds to half a peanut), depending on food preferences, or little black pebbles ( ∼ 0.01 m in diameter) and put on a sliding table in front of the subject. The sliding board consisted of grey polyvinylchloride (length 0.8 m, width 0.27 m, height 0.01 m) and was attached to a fixed polyvinylchloride table (length 0.8 m, width 0.38 m, height 0.01 m) by two drawer rails so that the sliding table could be moved horizontally. The sliding table was attached with an iron mount in front of a plastic panel (height 0.7 m, width 0.8 m). The plates were placed on the right and left side of the sliding table. Two holes (diameter 0.01 m, distance 0.3 m) in the plastic panel allowed the subjects to point with their fingers at the cups. It was possible to set up an occluder of grey plastic (length 0.8 m, height 0.3 m, thickness 0.03 m) in front of the panel so that the subject was not able to watch the baiting procedure. All sessions were videotaped with a digital video camera (Sony DCR-HC90E). Procedure Before each test condition, the subjects went through a familiarization phase to accustom them to the choice paradigm used in the following test condition. The procedure was the same in the familiarization and the corresponding test condition. The experimenter placed the two plates in the middle of the sliding table and baited every plate with the designated number of pieces (food or pebbles) behind an occluder, trying to avoid consistent arrangements of the choice stimuli. The occluder was removed and the experimenter waited until the animal paid attention (usually, they were already sitting in front of the table). Then the two plates were simultaneously moved in front of the two holes. After that the sliding table was pushed against the Plexiglas panel and the subject was allowed to choose. To avoid cueing the subject, the experimenter looked at the middle of the Plexiglas panel during the whole procedure (see also controls below). A choice was coded when the subject pointed with one finger to one of the locations through a hole in the screen. In the familiarization phase, the subjects were offered only two types of pairwise combinations (that is, 7 versus 1 and 8 versus 2) with 10–16 trials per session, one session per day. After reaching 80% correct responses within a session (always accomplished in the first or second session), the corresponding test session with different quantity combinations began. After the completion of each test condition, the subjects went through the new familiarization phase to introduce them to the paradigm of the next condition. In the test phase, we used the following conditions: Food: The experimenter put up the occluder in front of the plates and baited them with the designated quantity of food items (raisins or peanuts). Next, the occluder was removed, the plates were moved in front of the two holes and the sliding table was pushed against the Plexiglas panel. After the subject had made its choice, it received all the food items on the plate it had pointed at. Pebbles : The experimenter put up the occluder and placed the same number of food items (raisins or peanuts) underneath the plates as pebbles were placed onto the plates. Then the occluder was removed, the plates were moved in front of the holes, the table was pushed forward and the subjects could choose. The monkeys then received all food items under the plate they had pointed at. 'Food replaced' condition: The experimenter put up the occluder and placed the same number of food items (raisins or peanuts) underneath the plates as food items were placed onto the plates. For all baboons, raisins were put onto the plates and the same number of pieces of peanuts was put underneath. We can exclude that they may prefer peanuts to raisins and perform better because of this simple explanation, as some of the baboons did not want to take the peanuts near the end of the sessions, so we used raisins instead. In these trials, raisins were placed on top of the plates as well as underneath. The baboons performed equally in these trials and in the rest of these sessions. However, to exclude any inferences from using different food kinds as choice stimuli and reward, we always used the same kind of food as choice stimuli and reward for the macaques, thus peanuts and peanuts or raisins and raisins depending on the food preferences of each subject. After baiting, the occluder was removed, the plates were moved in front of the holes, the table was pushed forward and the subject could choose. The monkeys then received all peanuts or raisins, respectively, under the plate they pointed at. The subject's responses were initially coded live by the experimenter. To test for observer reliability 30% of all trials ( N =740) were independently scored by a second coder. The inter-observer reliability was excellent (Cohen's k: 0.98). Design Initially, we started the study with the baboons. Every subject received four sessions per condition (one session per day; except the baboon BH that received only two sessions in the 'Food replaced' condition and the baboon MC that participated only in the 'Food' condition because of motivational problems). One session consisted of 20 trials resulting in 80 trials per condition per animal, thus a total of 240 trials per animal (but only 200 for BH, and 80 for MC). Each session included five numeric differences (four experimental and one control difference), ranging from 0 to 4. Within each numeric difference, there were four trials with different quantities of items used ( Table 1 ). The sequence of the trials was balanced and the position of the larger quantity was counterbalanced across sessions. The baboons received the conditions in the following order: Food, Pebbles and 'Food replaced' condition. To exclude a learning effect across all conditions we repeated the initial 'Food' condition at the end. The baboons performed equally as in the first condition (70% correct), thus learning the different quantity combinations could not account for the differences in their performance in the other conditions. To test the consistency of the results found for the baboons, we repeated the test with long-tailed macaques. Every subject received two sessions (one session per day) in each of the three test conditions. One session consisted of 20 trials resulting in 40 trials per condition per animal, thus a total of 120 trials per animal. The design of the sessions was the same as for the baboons. To exclude any order effects, the order of the conditions was balanced across individuals. The control trials were conducted to examine whether subjects exhibited a laterality bias, that is, going on the same side on every trial. Furthermore, in the control trials of the 'Pebbles' condition, raisins were placed only under one plate to discover whether the subjects used other cues such as smell, sight or cues from the experimenter or the baiting procedure, which they did not (47.5% correct). Because it was suggested that the difference in performance might be due to the fact that in the Food condition, the choice stimuli had lesser associative strength because they changed in appearance while the items were fed to the monkeys (T Dickinson, personal communication), we ran a further set of control experiments with eight of the macaques (two subjects were excluded due to motivational problems). In the first control condition, all food items were taken away after the subject had made their choice ('Food away'), and then given to the monkeys while hidden in the experimenter's palm. In the second control condition ('Pebbles away'), we used pebbles as choice stimuli. After the subject made its choice, a pebble was removed each time when one of the food items underneath the plate was given to the monkey. To control for learning effects, we ran the initial 'Food' condition again. Overall, there was a slight increase in accuracy between the first and second sets of experiments in the 'Food' condition (74.1% correct). This increase was not significantly different ( P >0.2). Statistics We used a generalized linear mixed model implemented in the R statistical computing environment [32] . GLMM was implemented using the glmer function from the lme4 package [33] . We used species (2 levels), condition (3 levels), absolute magnitude of the difference (4 levels) and ratio (11 levels) as fixed factors and subject as random factor. A MCMC procedure was used to approximate the significance levels of the parameter estimates. In the additional control experiments, we only tested macaques, and compared the performance in the 'Food away' versus the 'Pebbles away' conditions. To test the effect of experience, we compared the performance of the macaques in the initial and repeated 'Food' condition. How to cite this article: Schmitt, V. & Fischer, J. Representational format determines numerical competence in monkeys. Nat. Commun. 2:257 doi: 10.1038/ncomms1262 (2011).